Probing the limits of gate-based charge sensing Quantum computation requires a qubit-specific measurement capability to readout the final state of individual qubits. Promising solid-state architectures use external readout electrometers but these can be replaced by a more compact readout element, an in situ gate sensor. Gate-sensing couples the qubit to a resonant circuit via a gate and probes the qubit’s radiofrequency polarizability. Here we investigate the ultimate performance of such a resonant readout scheme and the noise sources that limit its operation. We find a charge sensitivity of 37 μe Hz −1/2 , the best value reported for this technique, using the example of a gate sensor strongly coupled to a double quantum dot at the corner states of a silicon nanowire transistor. We discuss the experimental factors limiting gate detection and highlight ways to optimize its sensitivity. In total, resonant gate-based readout has advantages over external electrometers both in terms of reduction of circuit elements as well as absolute charge sensitivity. High-fidelity quantum state readout is a requirement for the implementation of a quantum computer. In semiconductor architectures, readout is typically performed via a separate, proximal charge sensor, in contrast to in situ gate-based readout [1] . To date, the most sensitive electrometers are the radiofrequency quantum point contact (rf-QPC) [2] , [3] , [4] and the radiofrequency single-electron transistor (rf-SET) [5] , [6] , [7] , providing charge sensitivities at the μe Hz −1/2 level [8] , [9] , [10] . However, the integration of these detectors add additional elements to the architecture, complicating scalability. Circuit quantum electrodynamics describes an alternative method to readout the state of a quantum system. The self-resonance of a high-frequency resonator is modified by the state-dependent polarizability of the quantum systems coupled to it. It allows readout via the dispersive and dissipative interaction between resonator and qubit. This technique has been demonstrated for superconducting qubits [11] , [12] , [13] , [14] and semiconductor charge [15] , [16] and spin qubits [17] , [18] . Outside the strong coupling limit of circuit quantum electrodynamics, resonant LC circuits have been coupled directly to the ohmic contacts of double quantum dots to readout their charge and spin state [19] , [20] , and to determine their complex admittance [21] . Furthermore, it has recently been demonstrated that the gates defining these quantum systems can also act as fast and sensitive readout elements, using the state-dependent polarizability as detection mechanism [1] . While the high-frequency polarizability of quantum systems is well understood in terms of Sisyphus resistance [22] , and state-dependent quantum or tunnelling capacitance [22] , [23] , [24] , [25] , the sensitivity of gate detection has only been reported at the me Hz −1/2 range for GaAs [19] , [26] . In other semiconductor materials, charge and spin readout have been achieved [27] , [28] , [29] , [30] , [31] , [32] and fast detectors have been demonstrated [33] , [34] , [35] but little progress has been made towards gate-based sensing [36] . More generally, the noise inherent to any fast-driven two-level system, akin to the cyclostationary noise [37] needs to be addressed in order to determine the fundamental limits of charge and phase sensitivity of resonant readout techniques. In the following, we demonstrate and benchmark a high-sensitivity gate-based charge sensor and calculate the sensitivity limits of resonant readout. The sensor alleviates the need for an external electrometer and simplifies the qubit architecture. It performs at unprecedented levels of sensitivity for gate-based readout, improving on previous semiconductor designs by two orders of magnitude [1] . The sensor is implemented on the gate electrode of a silicon tri-gate nanowire field-effect transistor (NWFET). By connecting the gate to a radiofrequency resonator we probe the charge state of a few-electron double quantum dot formed at the two top corners of the square NWFET channel. We obtain a charge sensitivity of δq =37 μe Hz −1/2 , owing to the strong capacitive coupling between the resonator and the quantum dots ( α = C g / C Σ=0.92 , where C g is the gate and C Σ is the total capacitance, respectively), which could be achieved in any nanowire geometry (for example, InAs or carbon nanotubes). Moreover, we explore the noise sources that limit resonant charge detection in the dispersive and dissipative regime and develop a model of the noise arising from the stochastic nature of electron tunnelling in fast-driven two-level systems. Our calculations show that the sensitivity is limited by a type of noise, which we call Sisyphus noise, that couples to the resonator’s natural frequency of oscillation. We use our model to determine the ultimate charge and phase sensitivity of gate-based detectors and predict that the latter have the potential to outperform rf-SETs. Device and measurement technique The device used here is a narrow channel silicon-on-insulator (SOI) nanowire transistor. A polycrystalline silicon top gate (length l =64 nm) wraps around three faces of the nanowire and is separated from the channel (width w =30 nm) by an oxide of 1.3 nm equivalent thickness offering a strong control over the channel electrostatics. The electric field exerted by the gate is strongest at the top most corners, where two gate faces meet. Owing to this so-called corner effect, electron accumulation in silicon NWFETs [38] happens first at the top most corners. In addition, potential irregularities along the transport direction [39] , [40] confine these corner channels creating a parallel double quantum dot as schematically displayed in Fig. 1a . We couple the double-dot to a resonant LC circuit via the top gate electrode as depicted in Fig. 1b and measure the reflected radiofrequency signal [6] , [19] , [41] . At the resonant frequency ( , C P is the detector’s stray capacitance) the magnitude ( γ ) and phase ( φ ) components of the reflected signal are sensitive to admittance changes of the device ( Fig. 1c ). Changes in the power dissipation in the system are captured in γ , whereas φ reflects susceptance changes because of tunnelling or quantum capacitance [1] , [21] , [24] . 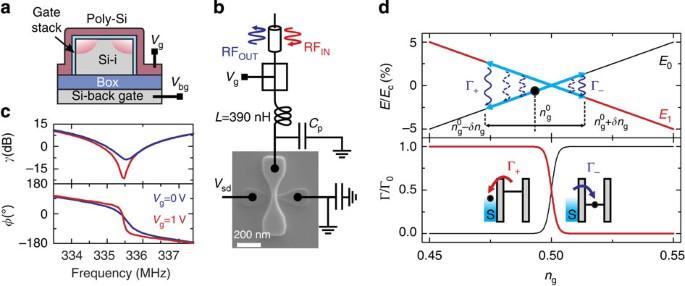Figure 1: Device and measurement set-up. (a) Sketch of the cross-section of the device perpendicular to the transport direction. Owing to the corner effect in silicon nanowire FETs and potential irregularities, a parallel few-electron double quantum dot system forms whenVgis biased just below threshold. (b) Electron micrograph of an equivalent device (l=64 nm,w=30 nm) embedded in a resonant tank circuit.Cpis the parasitic capacitance to ground andLa surface mount inductor.Vsd,VgandVbgare the DC voltages applied to the source, top gate and back gate, respectively. (c) Characterization of the reflectometry response in magnitude (top frame) and phase (bottom frame) for the OFF (Vg=0 V) and ON (Vg=1 V) state of the transistor. (d) Top panel: energy band diagram as a function of reduced gate voltageng. The initial detuning position is set byandδngis the amplitude of the RF excitation. Γ+(−)represents the tunnelling into (out of) the dot. Bottom panel: 3D–0D tunnel rates as a function ofngcalculated forEC=15 meV andT=100 mK. Figure 1: Device and measurement set-up. ( a ) Sketch of the cross-section of the device perpendicular to the transport direction. Owing to the corner effect in silicon nanowire FETs and potential irregularities, a parallel few-electron double quantum dot system forms when V g is biased just below threshold. ( b ) Electron micrograph of an equivalent device ( l =64 nm, w =30 nm) embedded in a resonant tank circuit. C p is the parasitic capacitance to ground and L a surface mount inductor. V sd , V g and V bg are the DC voltages applied to the source, top gate and back gate, respectively. ( c ) Characterization of the reflectometry response in magnitude (top frame) and phase (bottom frame) for the OFF ( V g =0 V) and ON ( V g =1 V) state of the transistor. ( d ) Top panel: energy band diagram as a function of reduced gate voltage n g . The initial detuning position is set by and δn g is the amplitude of the RF excitation. Γ +(−) represents the tunnelling into (out of) the dot. Bottom panel: 3D–0D tunnel rates as a function of n g calculated for E C =15 meV and T =100 mK. Full size image The origin of the gate-sensor signal can be understood in terms of electronic transitions in a fast-driven tunnel-coupled two-level system [42] . Here we consider inelastic charge tunnelling between the quantum dots and the leads. The levels E 0 (dot empty) and E 1 (dot full) are aligned at n g =0.5 as shown in Fig. 1d . The system is driven cyclically around a DC bias point with frequency ( f 0 ) comparable to the tunnel rate and amplitude . Here C g is the gate capacitance and V g and are the DC and RF gate voltage, respectively. Starting from the ground state at , the fast RF excitation δn g moves the system out of equilibrium to the right of the degeneracy point. The system is now in the excited state until it inelastically tunnels. The excess dissipated energy Δ E = E 0 − E 1 is then captured as a change in the total reflected power of the device. The dispersive signal may be detected when electrons on average tunnel out-of-phase with the rf cycle, generating an additional tunnelling capacitance contribution C t = α∂ ‹ ne ›/ ∂V g , where ‹ ne › is the average charge in the island. The mechanism has previously been studied in the context of Sisyphus dissipation for three-dimensional (3D) metallic islands [24] , [42] . Here we transfer the concept to confined systems with a 0D density of states coupled to 3D electron reservoirs. The corresponding tunnel rates are shown in the lower panel of Fig. 1d . A Fermi’s golden rule calculation yields the 3D–0D tunnel rates, where k B is the Boltzmann constant, T the temperature, Δ E ( t )= E c (1−2 n g ( t )) the time-dependent energy difference and is the normalized gate voltage. Γ 0 is the constant tunnel rate that establishes away from the degeneracy. In order to evaluate the performance of the gate sensor we first compare the results to standard direct current measurements. Fig. 2a shows the characteristic Coulomb diamonds where the electron occupancy is well defined. The onset of current happens at the diagonal lines marked by the green and red arrows indicating the alignment of the electrochemical levels of QD1 to the source and drain reservoirs, respectively (see Fig. 2b ). Moreover, we observe a shift of the high-current regions at the orange lines, which can be understood as a capacitive shift of the QD1 transport characteristics because of the loading of an electron on QD2. However, QD2 is only coupled to the source reservoir as depicted in Fig. 2b and cannot be measured in transport. 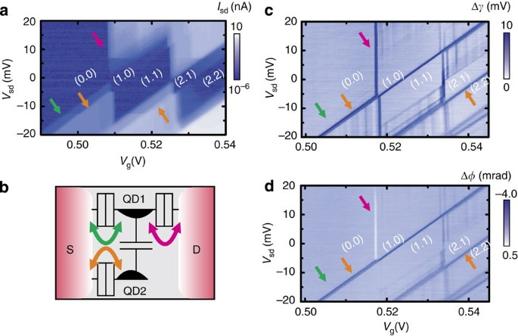Figure 2: DC/RF readout comparison. (a) Source-drain currentIsdas a function ofVgandVsdforVbg=2.4 V. The numbers (n,m) indicate the electron occupancy in in QD1 (n) and QD2 (m). The coloured arrows point to the onset of the transitions depicted inb. (b) Schematic diagram of a top view of the double-dot configuration. QD1 is tunnel-coupled to the drain (source) indicated by the magenta (green) arrows, while QD2 is only coupled to the source (orange arrow). Gate sensor magnitude response Δγ(c) and phase response Δφ(d) in the same bias region asa. Arrows indicate the same transitions as ina. Figure 2: DC/RF readout comparison. ( a ) Source-drain current I sd as a function of V g and V sd for V bg =2.4 V. The numbers (n,m) indicate the electron occupancy in in QD1 (n) and QD2 (m). The coloured arrows point to the onset of the transitions depicted in b . ( b ) Schematic diagram of a top view of the double-dot configuration. QD1 is tunnel-coupled to the drain (source) indicated by the magenta (green) arrows, while QD2 is only coupled to the source (orange arrow). Gate sensor magnitude response Δ γ ( c ) and phase response Δ φ ( d ) in the same bias region as a . Arrows indicate the same transitions as in a . Full size image The magnitude response of the gate sensor in the same voltage region as the DC transport experiment is presented in Fig. 2c . The signal outlines the edges of the charge-stable regions previously observed in the DC transport measurements. An important difference between the DC and RF measurements is observed, for example, at the QD2 charge transitions (orange arrows). The gate sensor magnitude response is enhanced when the electrochemical levels of dot QD2 and the source reservoir are aligned, demonstrating the possibility to detect charge transitions without the need of current flow or external charge sensors. The detector maintains its sensitivity at high V sd , as opposed to what is observed in 3D charge islands [24] . This additional feature stems from the independence of Γ ± on V sd (equation 1). In Fig. 2d we extract the dispersive contributions by analysing the phase response of the sensor. A change in the effective capacitance of the system because of electron tunnelling modifies the resonator’s resonant frequency and hence causes a phase shift at the sampling frequency ( f 0 ). The phase response relates to an effective change in the capacitance, Δ C , of the system given by Δ φ ≈− πQ Δ C / C P , where Q is the quality factor of the resonator. Analogously to the magnitude response, we observe this phase shift Δ φ at the edges of the conductive regions demonstrating dispersive readout of the charge state of a few-electron quantum dot system. Phase changes of the order of 1 mrad are easily resolved, translating into capacitance detection of ~1 aF, smaller than the ~fF quantum capacitance of strongly coupled quantum systems [25] . Experimental charge sensitivity We now move on to the experimental characterization of the gate sensor’s charge sensitivity. In Fig. 3a we show a typical transfer curve Δ γ − V g of the device comprising two charge transitions. We quantify the sensitivity by applying a small sinusoidal voltage (frequency f s ) to the top gate and monitoring the height of the sidebands in the frequency spectrum at f 0 ± f s . We perform this characterization at the point of maximum transconductance of the QD2 transition (red star) since there Γ 0 and f 0 are well matched. The inset i shows the optimal sideband signal obtained with an equivalent voltage amplitude Δ q =0.01e at f s =20 kHz. This results in a signal-to-noise ratio of 15.6 dB and a charge sensitivity of δq =37 μe Hz −1/2 given by ( [10] ), where B SA is the bandwidth of the spectrum analyser used to capture the signal. Owing to the strong capacitive coupling between the radiofrequency resonator and the quantum system ( α =0.92), our detector shows an improvement of two orders of magnitude as compared with recent GaAs gate sensors (6.3 me Hz −1/2 ) [1] . 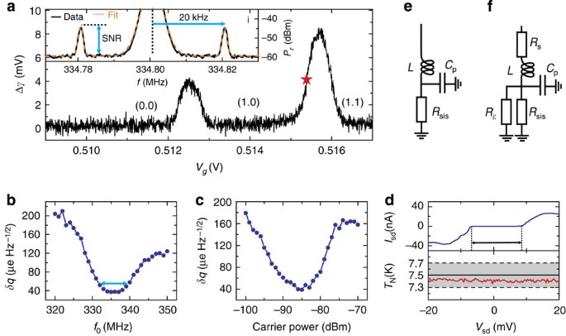Figure 3: Gate readout benchmark. (a) Typical transfer curve Δγ−Vgshowing two electron transitions.Vg=0.5125 V is the first electron on QD1 andVg=0.5157 V is the first electron on QD2. Inset (i) Sidebands at the point of maximum transconductance (Vg=0.5155 V) at 20 kHz and equivalent excitation amplitude of 0.01 e (solid black line) and fitted curve (dashed orange line). The measurement bandwidth isBSA=1 kHz. Charge sensitivity as a function of carrier frequency (b) and carrier power (c). The 3-dB bandwidth, equivalent to 8 MHz, is indicated by the blue arrow. (d) Top panel: source-drain current (Isd) as a function of source-drain voltageVsdthrough a blockaded region atVg=0.58 V. Bottom panel: noise temperature as a function of source-drain voltage measured at the resonant frequency with a resolution bandwidth of 1 MHz (red solid line). No rf excitation is applied during this measurement. The grey band indicates the calibrated noise temperature of the cryogenic amplifier,TN=7.5±0.2 K. Lossless (e) and lossy (f) impedance matching circuits.Rsisis the Sisyphus resistance of the device,Rsis the inductor equivalent series resistance andRεis the equivalent dielectric loss of the resonator. Figure 3: Gate readout benchmark. ( a ) Typical transfer curve Δ γ − V g showing two electron transitions. V g =0.5125 V is the first electron on QD1 and V g =0.5157 V is the first electron on QD2. Inset (i) Sidebands at the point of maximum transconductance ( V g =0.5155 V) at 20 kHz and equivalent excitation amplitude of 0.01 e (solid black line) and fitted curve (dashed orange line). The measurement bandwidth is B SA =1 kHz. Charge sensitivity as a function of carrier frequency ( b ) and carrier power ( c ). The 3-dB bandwidth, equivalent to 8 MHz, is indicated by the blue arrow. ( d ) Top panel: source-drain current ( I sd ) as a function of source-drain voltage V sd through a blockaded region at V g =0.58 V. Bottom panel: noise temperature as a function of source-drain voltage measured at the resonant frequency with a resolution bandwidth of 1 MHz (red solid line). No rf excitation is applied during this measurement. The grey band indicates the calibrated noise temperature of the cryogenic amplifier, T N =7.5±0.2 K. Lossless ( e ) and lossy ( f ) impedance matching circuits. R sis is the Sisyphus resistance of the device, R s is the inductor equivalent series resistance and R ε is the equivalent dielectric loss of the resonator. Full size image In addition, we study the dependence of δq on carrier frequency and carrier power. Figure 3b shows an optimal δq for a carrier at 335 MHz with a detection bandwidth B of 8 MHz (blue arrow) implying a loaded Q-factor of 42. The optimal excitation power is found to be −85 dBm, which is equivalent to and a RF amplitude δn g =0.03 ( Fig. 3c ) 50 times larger larger than k B T / E C . Combined with the broad detection bandwidth, the two order of magnitude improvement of sensitivity will now allow single-shot readout of electron spins in semiconductor nanostructures, where T 2 times are at least of the order of μs [31] , [43] , [44] . In fact, our gate-based sensor allows submicrosecond detection with an rms charge noise (ref. 6 ) of ≃ 0.1 e. As a whole, these results demonstrate that gate-based readout is a sensitive alternative to the best reported rf-QPCs (ref. 9 , and normal and superconducting rf-SETs (1 and 0.9 μe Hz −1/2 ) (refs 8 , 10 ). The sensitivity of rf-SETs is limited by shot noise because of the stochastic nature of the current through the tunnel barriers [45] . Similarly, resonant readout techniques are in theory limited in their sensitivity by the noise that arises because of the fast drive exerted on the system. A discussion of this type of cyclostationary noise follows in the next section. Here we discuss external factors limiting the gate sensor performance. In Fig. 3d we experimentally characterize the noise temperature of the system at the resonant frequency as a function of V sd : The top panel shows the source-drain current across a Coulomb blockade region; the bottom panel displays the system’s noise temperature, T N in the same region. T N remains constant independent of the device’s current level and coincides with the noise temperature of the cryogenic amplifier, 7.5±0.2 K highlighted in grey (The amplifier noise was calibrated using shot noise thermometry according to ref. 46 . ). We conclude that the noise, and hence also the sensitivity of the gated-based charge sensor presented here, is experimentally limited by the noise level of the first amplification stage and is independent of I sd as opposed to shot-noise-limited rf-SET detectors [45] , [47] . Furthermore, degradation of the detector’s sensitivity can arise from external sources of dissipation such as losses in the resonator components. We model these effects using an equivalent lumped-element circuit (see Fig. 3e,f ) consisting of the device’s typical Sisyphus resistance ( R sis =300 kΩ), the equivalent series resistance of the inductor ( R s =5.2 Ω) and the equivalent dielectric loss ( R ε =16 kΩ) because of losses in the PCB board and the geometrical capacitance of the device (see Supplementary Fig. 1 and Supplementary Note 1 ). Losses because of the inductor account for a detrimental 10% on sensitivity, which could be improved by the use of a superconducting on-chip inductor. Dielectric losses account for 67% reduction, which could be alleviated by using lower loss PCB boards and optimizing the sample geometry to minimize the parasitic geometrical capacitance. For a lossless circuit as shown in Fig. 3e , we predict that the measured sensitivity could be lowered to 10 μe Hz −1/2 . Finally, an improvement of δq could be achieved if the resonant circuit were designed to match the high Sisyphus impedance of the device, for example, using superconducting transmission lines to make a stub matching network [48] . We estimate that using this technique a minimum charge sensitivity of 0.9 μe Hz −1/2 could be achieved. Sisyphus model and comparison to experiment We now turn to a theoretical description of resonant charge readout. It is substantially different from rf-SETs where the largest contribution to the reflected power comes from the modulation of its differential conductance. In resonant readout schemes single-electron tunnelling is directly coupled to the frequency of the rf-drive and therefore a frequency-dependent noise spectrum is expected. To calculate the fundamental noise that limits resonant charge detection we develop a model of the correlation of the power and phase fluctuations in a fast-driven two-level system. In the following we neglect the back action of photon shot noise since our coupled resonator-qubit system is in the weak-coupling regime [49] . We first focus on the dissipative components associated with fast electronic transitions. We present in the following a numerical calculation of the instantaneous dissipated power, P ( t ), due to the rf excitation, the corresponding spectral density of the fluctuations in dissipated power, S pp , and the charge sensitivity, δq , using experimental parameters obtained earlier. The dynamics of power dissipation are given by a master equation [42] . For the 0D–3D tunnel rates (equation (1)) it reduces to solving the differential equation, where P 1 is the probability of the electron being in the dot. Solving equation (2) for P 1 ( t ) we obtain the instantaneous dissipated power as well as its average, ‹ P ›, over one period , which is shown in Fig. 4a as a function of DC offset . It is displayed for several tunnel rates, using the optimal RF excitation δn g =0.03. The most power is dissipated when the system is biased at the charge instability and no dissipation occurs for , as expected. The change in average power dissipation, , is maximum at . 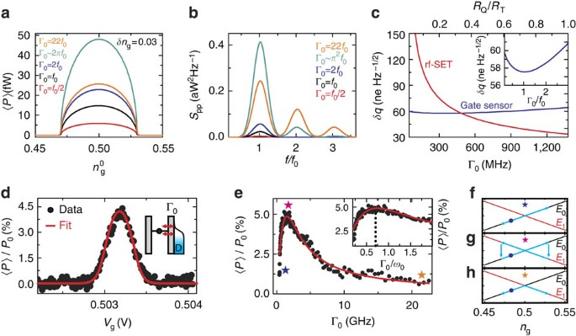Figure 4: Sisyphus power dissipation and ultimate charge sensitivity. (a) Calculated average power dissipation as a function of reduced gate voltagefor different tunnel rates Γ0and reduced rf amplitudeδng=0.03. (b) Power spectral density of the power noise,Spp, as a function of normalized frequencyf/f0for several tunnel rates at. (c) Gate-based noise-limited charge sensitivity as a function of tunnel rate (blue line). rf-SET ultimate sensitivity as a function of the ratio between the quantumRQand tunnel resistanceRT(red trace) from ref.47.RT=2kBT/e2Γ0at ΔE=0. Inset: zoom-in close to the resonant frequency. The best sensitivity is achieved at the resonant frequencyf0.T=100 mK andEC=15 meV throughout the calculations. (d) Experimental (black dots) and simulated data (red solid line,δng=0.0125,T=1 K and Γ0=1 GHz) of the ratio of dissipated power due to the cyclical exchange of electrons ‹P› and total power dissipated by the resonatorP0as a function ofVg. (e) Maximum ‹P›/P0as a function of tunnel rate Γ0for the transition indicated by the magenta arrow inFig. 2c. (Inset) Zoom-in to the region Γ0≈ω0. The red solid line is a fit according to equation 4. Schematic diagrams referring to the no tunnelling (f), inelastic tunnelling (g) and elastic tunnelling regimes (h). Figure 4: Sisyphus power dissipation and ultimate charge sensitivity. ( a ) Calculated average power dissipation as a function of reduced gate voltage for different tunnel rates Γ 0 and reduced rf amplitude δn g =0.03. ( b ) Power spectral density of the power noise, S pp , as a function of normalized frequency f/f 0 for several tunnel rates at . ( c ) Gate-based noise-limited charge sensitivity as a function of tunnel rate (blue line). rf-SET ultimate sensitivity as a function of the ratio between the quantum R Q and tunnel resistance R T (red trace) from ref. 47 . R T =2 k B T / e 2 Γ 0 at Δ E =0. Inset: zoom-in close to the resonant frequency. The best sensitivity is achieved at the resonant frequency f 0 . T =100 mK and E C =15 meV throughout the calculations. ( d ) Experimental (black dots) and simulated data (red solid line, δn g =0.0125, T =1 K and Γ 0 =1 GHz) of the ratio of dissipated power due to the cyclical exchange of electrons ‹ P › and total power dissipated by the resonator P 0 as a function of V g . ( e ) Maximum ‹ P ›/ P 0 as a function of tunnel rate Γ 0 for the transition indicated by the magenta arrow in Fig. 2c . (Inset) Zoom-in to the region Γ 0 ≈ ω 0 . The red solid line is a fit according to equation 4. Schematic diagrams referring to the no tunnelling ( f ), inelastic tunnelling ( g ) and elastic tunnelling regimes ( h ). Full size image With respect to tunnel rates, ‹ P › peaks at Γ 0 =2 πf 0 showing a way to maximize the detector response. This can be understood from the analytical approximation given in equation (4), where Γ ± is expanded around to the first order of δn g . Note that this approximation is only valid for excitations δn g ≪ k B T / E C . The numerical solution P 1 ( t ) of equation (2) (see Supplementary Note 3 ), furthermore, allows us to calculate the power fluctuations around the mean value and subsequently their power spectral density, S pp (see Supplementary Note 2 ). The results are shown in Fig. 4b as a function of reduced frequency f / f 0 for several Γ 0 at . At the point of maximum sensitivity the power noise is maximum at frequencies that match the excitation frequency f 0 and its harmonics. As a whole, these calculations show a new type of frequency-periodic noise, the Sisyphus noise, in which the stochastic nature of electron tunnelling is directly coupled to the resonator’s natural frequency of oscillation. However, signal and noise frequency decoupling could be achieved at the degeneracy point (See Supplementary Fig. 2 ). Knowledge of the Sisyphus noise and the change in average power dissipation allows us now to calculate the charge sensitivity in units of e Hz −1/2 . The result is presented in Fig. 4c (main panel and inset). In blue we show the charge sensitivity as a function of tunnel rate for S pp ( ω )= S pp (2 πf 0 ) and , which corresponds to the experimental situation presented earlier. For our experimental set-up and a range of tunnel rates, the fundamental limit of dissipative rf charge read-out is δq ≲ 70 ne Hz −1/2 . As can be seen from the inset of Fig. 4c , the best charge sensitivity occurs for matching tunnel rate and excitation frequency. Adjusting Γ 0 and f 0 may thus be a route to obtain the best sensitivity, although experimental constraints such as the resonant circuit, that is, f 0 , will set a practical limit. We benchmark our detector’s ultimate sensitivity against that of rf-SETs predicted in ref. 47 (red trace in Fig. 4c ). A direct comparison is made considering the tunnel resistance equivalent R T =2 k B T / e 2 Γ 0 , which sets the same tunnel rate at Δ E =0 for both cases. Comparing both curves, we find that rf-SETs exhibit a better fundamental charge sensitivity at high tunnel rates, whereas our rf gate sensor performs favourably at low Γ 0 , that is, for highly resistive tunnel barriers, which is the usual scenario of quantum dots in the few-electron regime. We confirm the accuracy of our simulations by comparing them to experimental data. In Fig. 4d we plot the ratio of power dissipated in the device, ‹ P ›, and total dissipated power in the resonator, P 0 , as a function of V g across a charge transition point. The lineshape of the peak presents a cosh 2 dependence (see equation 4) and is reproduced by our numerical simulations. Furthermore, we compare the experimental and theoretical dependence of ‹ P › on tunnel rates. In the cyclical exchange of electrons between dot and electron reservoirs, ‹ P › depends on the ratio of the drive frequency ω 0 =2 πf 0 and the tunnel rate Γ 0 , as seen in equation 4. While ω 0 is fixed in the experiment, Γ 0 can be tuned by changing the profile of the tunnel barriers. This is controlled electrostatically by means of the back gate voltage V bg . The effect of changing tunnel rates on the detector’s response is demonstrated in Fig. 4e , where we plot the maximum ‹ P ›/ P 0 arising from an exchange of electrons between QD1 and the drain reservoir (magenta arrow in Fig. 2c ) as a function of Γ 0 (see Supplementary Fig. 3 ). The data are well fitted by our model (red line), and may be understood as follows. At low tunnel rates no additional power is dissipated in the device since there is insufficient time for electrons to tunnel at the rf-drive timescale ( Fig. 4f ). Equally, at high tunnel rates no power is dissipated as electron tunnelling is elastic ( Fig. 4h ). However, when Γ 0 ≈0.75 ω 0 , power dissipation is maximized as on average tunnelling happens inelastically at the end of the rf cycle ( Fig. 4g ). The deviation from the expected Γ 0 = ω 0 at which the dissipated power is maximized (see equation 4) could be a results of a small coupling asymmetry to the source and drain reservoirs of QD1 (see Supplementary Note 4 ). Dispersive readout We now move on to the analysis of dispersive readout and the limits of gate-based phase sensing. Here the change in the probability of the electron being in the dot because of the rf-drive generates a tunnelling capacitance term given by, which in turn generates a phase shift Δ φ ( t ) ∝ − C t ( t ). We confirm our calculations in Fig. 5a by comparing experimental data to the theoretical average phase shift ‹Δ φ ›. Similarly to the average power dissipation, the phase response peaks at the degeneracy point and the change is maximum close to . C t is always positive independently of T and Γ 0 and hence ‹Δ φ › remains negative, which indicates that on average electron tunnelling leads the rf excitation unless the transient behaviour of the system is probed (see Supplementary Note 2 ). 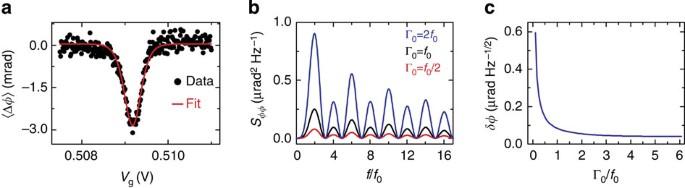Figure 5: Sisyphus phase response and ultimate phase sensitivity. (a) Experimental data (black dots) and simulation (red solid line) of the average phase shift because of the cyclical exchange of electrons ‹ΔΦ› as a function ofVg. The simulation was performed atδng=0.0125,T=1.4 K and Γ0=380 MHz. (b) Power spectral density of the phase noise,Sφφ, as a function of normalized frequencyf/f0for several tunnel rates at. (c) Noise-limited phase sensitivity as a function of reduced tunnel rate. Lowest phase sensitivity is found for high tunnel rates Γ0>>f0. For all calculations leading to results inb,cT=100 mK andEC=15 meV. An analytical solution of equation (6) for δn g ≪ k B T / E C confirms this result, Figure 5: Sisyphus phase response and ultimate phase sensitivity. ( a ) Experimental data (black dots) and simulation (red solid line) of the average phase shift because of the cyclical exchange of electrons ‹ΔΦ› as a function of V g . The simulation was performed at δn g =0.0125, T =1.4 K and Γ 0 =380 MHz. ( b ) Power spectral density of the phase noise, S φφ , as a function of normalized frequency f/f 0 for several tunnel rates at . ( c ) Noise-limited phase sensitivity as a function of reduced tunnel rate. Lowest phase sensitivity is found for high tunnel rates Γ 0 >> f 0 . For all calculations leading to results in b , c T =100 mK and E C =15 meV. Full size image In contrast to the average power dissipation, ‹Δ φ › does not peak at the resonant frequency and tends to a constant value for large Γ 0 . This offers a way to maximize the dispersive signal while reducing the excess power dissipation. The phase noise spectral density associated with the phase fluctuations is presented in Fig. 5b . It is maximum at multiple of 2 f 0 with odd harmonics predominantly contributing to the noise spectrum. This can be explained from the time symmetry of the tunnelling capacitance: C t ≈tan( ω 0 t ) is an odd function of time and periodic in 1/2 f 0 (see Supplementary Note 3 ). Signal and noise are hence decoupled in frequency space offering an opportunity for high-sensitivity phase detection. The detector’s ultimate phase sensitivity, δφ , is calculated in the same way as its charge counterpart (see equation (5)) as the ratio of phase noise and change in average phase . It is plotted in Fig. 5c as a function of reduced tunnel rate at bias and frequency ω =2 πf 0 . In tune with ‹ φ › the phase sensitivity has no minimum at f 0 but approaches a low constant value at high tunnel rate. For parameters corresponding to our set-up the fundamental limit of phase sensitivity is δφ ≲ 0.04 μrad Hz −1/2 for tunnel rates Γ 0 >> f 0 . Fast gate-based phase detection is thus suitable for systems with transparent tunnel barriers, but performs also well at moderate tunnel rates. This result compares favourably to phase detection based on cooper-pair transistors, which provides sensitivities of the order of 1 μrad Hz −1/2 (ref. 50 ). In conclusion, we have reported the high-sensitivity resonant charge readout of a few-electron double quantum dot in silicon and studied its experimental and theoretical limits. The ultimate sensitivity of resonant readout, set by the Sisyphus noise arising in fast-driven two-level systems, is comparable to the best rf-SET charge sensors at an equivalent measurement bandwidth. Resonant gate-sensing can be introduced in all semiconductor materials where a strong coupling between gate and qubit can be engineered. A high-sensitivity in situ readout can then be achieved by eliminating sources of excess dissipation such as losses in the inductor and substrate, providing a resonant circuit matching the high-gate impedance, and matching rf-excitation frequency to the electron tunnel rates. Resonant gate-sensing therefore offers a competitive alternative to external charge detectors. The combination of high sensitivity and large bandwidth will allow for single-shot readout of electron spins in semiconductors. Moreover, the flexibility of this technique, which eliminates the need for external sensor elements, opens up a window for high-fidelity, high-integration qubit architectures. Device fabrication The nanowire transistors used in this study were fabricated on SOI substrates with a 145-nm buried oxide. The silicon layer is patterned to create the nanowires by means of optical lithography, followed by a resist trimming process. For the gate stack, 1.9-nm HfSiON capped by 5 nm TiN and 50 nm polycrystalline silicon were deposited, leading to a total equivalent oxide thickness of 1.3 nm. The Si thickness under the HfSiON/TiN gate is 11 nm. After gate etching, a SiN layer (thickness 10 nm) was deposited and etched to form a first spacer on the sidewalls of the gate. 18-nm-thick Si raised source and drain contacts were selectively grown before the source/drain extension implantation and activation annealing. Then a second spacer was formed and followed by source/drain implantations, activation spike anneal and salicidation (NiPtSi). Measurement set-up Measurements were performed at the base temperature of a dilution refrigerator. Radiofrequency reflectometry was performed at 335 MHz by embedding the sample in a resonant LC circuit formed by a surface mount inductor (390 nH) and the device’s parasitic capacitance to ground (500 fF). After low temperature and room temperature amplification, the reflected signal was fed into a quadrature demodulator, yielding the signal’s quadrature and in-phase component from which magnitude γ and phase φ are calculated. Numerical calculations P 1 ( t ) and all subsequent derivatives such as P ( t ) or Δ φ ( t ) are finite time series in the numerical calculations. P 1 ( t ) was obtained by solving equation (2) numerically for a range of parameters corresponding to experimental constraints, namely f 0 =335 MHz, T =100 mK, E C =15 meV and δn g =0.03, at equal time steps in the interval . The averages ‹ P › and ‹Δ φ › are taken over one full period. Owing to the finite time series nature of all variables no autocorrelation is necessary, but S pp ( S φφ ) can be calculated immediately from the power (phase) fluctuations: S XX ( ω )=(Δ t ) 2 f 0 |∑ n ( X ( n Δ t )−‹ X ›) × e − iωn | 2 . How to cite this article : Gonzalez-Zalba, M. F. et al . Probing the limits of gate-based charge sensing. Nat. Commun. 6:6084 doi: 10.1038/ncomms7084 (2015).